Violation of a Leggett–Garg inequality with ideal non-invasive measurements The quantum superposition principle states that an entity can exist in two different states simultaneously, counter to our 'classical' intuition. Is it possible to understand a given system's behaviour without such a concept? A test designed by Leggett and Garg can rule out this possibility. The test, originally intended for macroscopic objects, has been implemented in various systems. However to date no experiment has employed the 'ideal negative result' measurements that are required for the most robust test. Here we introduce a general protocol for these special measurements using an ancillary system, which acts as a local measuring device but which need not be perfectly prepared. We report an experimental realization using spin-bearing phosphorus impurities in silicon. The results demonstrate the necessity of a non-classical picture for this class of microscopic system. Our procedure can be applied to systems of any size, whether individually controlled or in a spatial ensemble. There is a stark contrast between the way we think of the microscopic world (which is well described by quantum physics) and the way we experience the everyday macroscopic world (which appears to follow altogether more intuitive rules). There have been a number of proposals for experimental tests which pit quantum physics against alternative views of reality: for example the theorems of Bell [1] and of Kochen and Specker [2] . Corresponding laboratory tests have been performed and to date support the necessity of quantum physics. But even if a quantum description of the microscopic world is necessary, we face the equally profound question of understanding the relationship between the quantum world and our familiar classical experience. Some thinkers, such as Penrose, suggest that there are as yet undiscovered physical laws, which prevent superposition of 'macroscopic' states [3] . Most physicists would agree that sufficiently large objects (such as the moon) must indeed 'be there' when nobody looks. The Leggett–Garg inequality [4] was developed in order to address this question. The protocol may be applied to systems of arbitrary size, thus theories which hold that quantum theory breaks down at some particular scale can be experimentally tested. Limited variants of the Leggett and Garg (LG) test have been reported for microscopic objects such as photons [5] , [6] or nuclear spins [7] and for the larger superconducting 'transmon' system [8] . The approach presented here represents the first implementation of LG's powerful 'ideal negative result' measurement procedure. We describe a general protocol for such measurements, introducing an ancillary system [9] , which acts as a local measuring device. Importantly we can account for imperfect preparation of the measuring device through a quantity, which we call 'venality'. We find that at some finite venality (typically corresponding to a thermal threshold) the LG test becomes possible. Our procedure can be employed for any physical system where a suitable ancilla can be adequately initialized; it thus provides a test for a system of any size, whether addressed as part of a spatial ensemble or controlled individually. For a given system with two suitably defined states, our protocol provides the opportunity to invalidate the conjunction of the following two beliefs: macrorealism (MR)—the system is always in one of its macroscopically distinguishable states; and non-invasive measurability (NIM)—it is possible in principle to determine the state of the system without altering its subsequent evolution. A quantum physicist will typically reject NIM, but crucially the test requires only that the macrorealist accept it [10] , [11] . In a test of the above assumptions, a compelling argument for the non-invasiveness of the measurements should be made in a language acceptable to a macrorealist. Leggett–Garg inequality violations that have been reported with weak measurements [5] , [6] , [8] employ a measurement procedure which may ultimately fail to convince a macrorealist that the measurements are indeed non-invasive. Proposals for experimentally determining the invasiveness of each measurement exist [12] , but we make use of Leggett and Garg's arguments for the non-invasiveness of an 'ideal negative result' measurement scheme. Other experiments have been performed [7] , [8] that use the assumption of 'stationarity' [13] , [14] , [15] . This assumption severely narrows the class of macrorealist theories which are put to the test (please see Supplementary Methods ); we do not make this assumption and hence our method tests a wider class of theories. We employ a method that equips a two level system with a local measuring device: another two-level system [9] . We refer to the system being tested as the 'primary system' and the associated measuring device as the 'ancilla'. We consider how macrorealists might approach an imperfectly prepared measuring device, showing that even an 'adversarial' macrorealist who makes the most extreme assumptions about the effects of invasive measurements must nevertheless expect certain constraints. Quantum physics predicts that under certain conditions such constraints can still be violated. We show that although the primary system may be in a totally mixed state, the degree to which the ancilla is correctly initialized directly affects one's ability to violate the constraint. We implement our protocol experimentally using an ensemble of nucleus–electron spin pairs in phosphorus-doped silicon. The results comprehensively rule out a large range of classical descriptions for this class of system, which although microscopic represents an important step towards performing rigorous tests on more macroscopic systems. Three core experiments Consider the primary system's two states of interest labelled by ↑ or by ↓ undergoing arbitrary dynamics governed by a process labelled U . If the system is probed at distinct times with a measurement which distinguishes one state from the other ( Fig. 1a ), the degree to which the state of the system correlates with itself at the different times may be quantified. The two-time correlator K ij =〈 Q ( t i ) Q ( t j )〉 is the expected value of the product of the measurement outcome of the observable Q at time t i and at time t j . If Q ∈ {+1, −1} for ↑, ↓ respectively, and as the correlator is an average, we have −1≤ K ij ≤1. Calculating this quantity is straightforward: one simply measures at t i , waits, and measures again at t j multiplying the results together to compute Q ( t i ) Q ( t j ). One then averages over many instances of the experiment either by repeating it many times, or by employing an array of many identical systems, as in a recent test of non-contextuality [16] . Although in a spatial ensemble one has no access to individual elements, because of the ancillary nature of the measuring qubit (each element of the ensemble is coupled to its own), the test may still be performed. 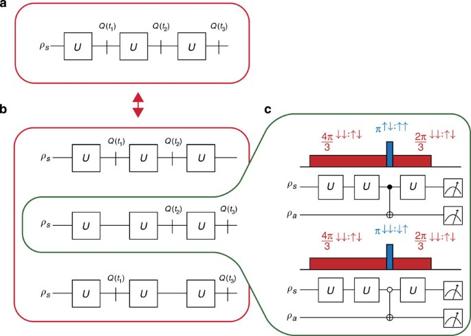Figure 1: Our full implementation of the LG test requires six subexperiments. If the measurements are non-invasive, the outcome statistics ofa, a single ideal experiment (where all measurements are made in each run) will match those ofb, a set of three core experiments (where only two measurements are made in each run). The actual lab implementation for the second of the three core experiments is shown in panelc. Shown in colour are the corresponding pulses applied to our experimental coupled-spinsystem. The primary system is driven with radio-frequency pulses (red areas), and the cnot and anti-cnot operations are each applied with a single selective microwave frequency pulse (blue areas). The other two core experiments are similarly resolved into a pair of complimentary subexperiments. Figure 1: Our full implementation of the LG test requires six subexperiments. If the measurements are non-invasive, the outcome statistics of a , a single ideal experiment (where all measurements are made in each run) will match those of b , a set of three core experiments (where only two measurements are made in each run). The actual lab implementation for the second of the three core experiments is shown in panel c . Shown in colour are the corresponding pulses applied to our experimental coupled-spin system. The primary system is driven with radio-frequency pulses (red areas), and the cnot and anti-cnot operations are each applied with a single selective microwave frequency pulse (blue areas). The other two core experiments are similarly resolved into a pair of complimentary subexperiments. Full size image Now consider a family of three experiments, each one beginning with a primary system in an identical initial state ρ s and evolving under identical conditions governing the dynamics of the state. In the first experiment measurements are made at t 1 and t 2 to determine K 12 . In the same way the second and third experiments are used to determine K 23 and K 13 ( Fig. 1b ). We then evaluate the 'Leggett–Garg Function' [4] : Any macrorealist theory according to which the measurements Q are non-invasive must predict f ≥0. This is true regardless of how the theory distributes probability arbitrarily among classical trajectories of the primary system (the assumption of 'induction' is required, see ref. 17 , Supplementary Methods ). In contrast, according to quantum physics, f is negative for suitably chosen time evolution operator U . Ideal negative result measurements Following Leggett [4] , [17] , [18] , [19] , we implement measurements of Q which, by exploiting MR, are 'extremely natural and plausible' [4] candidates for non-invasiveness. Imagine a measuring device that is physically incapable of interacting with a system in state ↑, but that will (possibly invasively) detect a system in state ↓. Suppose we apply this detector to our system and it does not 'click'; the macrorealist infers the system is in state ↑, and was in this state immediately before measurement—but this information is obtained without any interaction. Switching to a complementary measuring device that perceives only the ↑ state allows one to obtain the full set of data non-invasively, as long as one always abandons all experiments where the detector clicks. One must acknowledge that it is impossible to ensure that the measurement apparatus does not couple to and disturb some other, hidden, degrees of freedom. One cannot exclude macrorealist theories involving interactions between hidden parts of the system and detector (which in our case would have to occur even during a null measurement event). This is a general point applying to any LG test: one can only address a subclass of macrorealist theories which hold that such irremediable hidden degrees of freedom either do not exist, or are not relevant. The use of two detector configurations means that the three experiments introduced previously are each further resolved into a pair of experiments, one for non-invasive measurement of ↑, and one for ↓ ( Fig. 1c ). We utilize either a CNOT gate (which will flip the state of the ancilla if the control, that is, the primary system, is in ↓) or use an anti-CNOT gate (which will flip the state of the ancilla qubit if the primary is in ↑; Fig. 1 ), in each case post selecting experimental runs where the gate was not triggered ( Supplementary Methods ). The second, final measurement in each experiment need not be implemented non-invasively, as the subsequent dynamics are irrelevant. Note that it is important that the physical implementation of the CNOT (and anti-CNOT) operation is such that the primary system receives no perturbation when it is in the state associated with a null result. Here we set . As long as the ancilla is correctly initialized, the quantum prediction is K ij =cos ( θ ) independent of ρ s and hence which takes when the value f =−0.5 for θ =2 π /3, violating the inequality f ≥0 predicted under MR ∩ NIM. Arguments constraining the macrorealist to non-negative values for f also do not depend on the primary system's initial state. Corrupt ancillas For any protocol employing a measurement ancilla, its initialization is of fundamental importance. A macrorealist regards an imperfectly prepared primary-ancilla qubit pair as a statistical mixture of the four states |↓↓〉, |↓↑〉, |↑↓〉, |↑↑〉 and similarly a quantum physicist describes the initial state as a density matrix diagonal in the | system 〉| ancilla 〉 basis. According to quantum physics, an incorrectly initialized ancilla will give rise to a change in the sign of the correlator. To the macrorealist it will give a false indication that the measurement had been non-invasive, allowing a potentially corrupt element through the post selection. We define the venality ζ as the fraction of the ensemble for which the ancilla is incorrectly prepared. Quantum physics predicts that each K ij generalizes to (1− ζ ) K ij − ζK ij , leading to We identify two macrorealist attitudes pertaining to the effect of an invasive measurement. A 'moderate' view is that any invasively perturbed systems act in a random way, and hence average to produce zero net correlation. Then K ij →(1− ζ ) K ij and hence with g = K 12 + K 23 + K 13 and g ≥−1 for a macrorealist, Note f is still constrained to be non-negative. An 'adversarial' view is that invasively perturbed elements will, by some unidentified process, act in such a manner as to minimize f . Consequently K ij →(1− ζ ) K ij − ζ hence that This is the most aggressive stance available to a macrorealist. 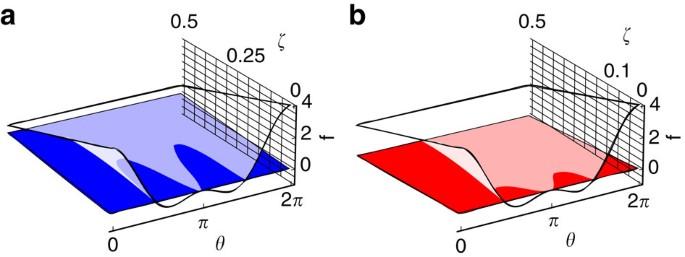Figure 2: The bounds on the LG inequality for quantum mechanical and macrorealist models depend on the venality in the experiment. Plots of the quantum mechanical prediction (white) and lower bound of a modified inequality for thea, moderate (blue) andb, adversarial (red) macrorealist attitudes as a function of the angleθand the venalityζ. Where the quantum prediction dips below the macrorealist bound it is in principle possible to invalidate the macrorealist stance. Note the critical value ofζ=0.25 andζ=0.1 above which one cannot exclude macrorealism for the moderate and adversarial approaches, respectively. The relevant thresholds are plotted in Figure 2 , showing that minimizing ζ is crucial for a successful experiment. Figure 2: The bounds on the LG inequality for quantum mechanical and macrorealist models depend on the venality in the experiment. Plots of the quantum mechanical prediction (white) and lower bound of a modified inequality for the a , moderate (blue) and b , adversarial (red) macrorealist attitudes as a function of the angle θ and the venality ζ . Where the quantum prediction dips below the macrorealist bound it is in principle possible to invalidate the macrorealist stance. Note the critical value of ζ =0.25 and ζ =0.1 above which one cannot exclude macrorealism for the moderate and adversarial approaches, respectively. Full size image Experimental implementation To demonstrate an experimental violation of these inequalities, we consider an ensemble of phosphorus donors in silicon, consisting of electron–nuclear spin pairs. Here the nuclear spin is the primary system, whereas the electron is the measurement ancilla. In the high-field limit, the eigenstates of this spin —spin system are precisely the four product spin states. In thermal equilibrium, and ignoring the weak polarization of the nucleus, these states are populated according to the Boltzmann distribution, where the spin states are in the ratio α :1 for . Here B =3.357 T is the magnetic field, g is the electron spin's g -factor, μ is the Bohr magneton, k B is Boltzmann's constant and T is the temperature. The electron and nuclear spin are coupled through a 117.5 MHz hyperfine interaction, which distinguishes each individual |↑〉 : |↓〉 transition. The electronic (nuclear) transitions can be individually addressed using selective microwave (radio-frequency) pulses. The unitary nuclear rotation U may be performed in a manner which is conditional on the system being in the 'correct' ancilla state ↓ (as a refinement of the circuit illustrated in Fig. 1c ) because the post selected data will always correspond to the unitary operation U having been applied. 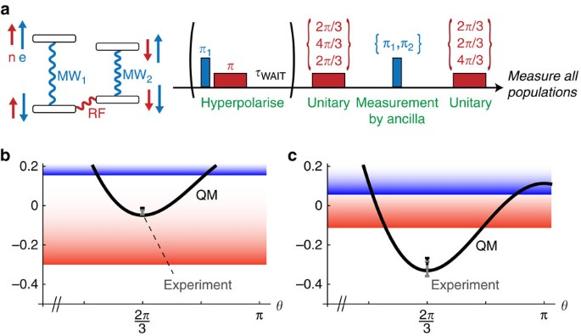Figure 3: Experimental values for the LG function are compared with bounds from quantum mechanics and macrorealist theories. (a) The populations of the four system-ancilla (nucleus–electron) states are manipulated with microwave and radio-frequency radiation. The experimentally determined value of the Leggett–Garg function at a static field ofB=3.357 T is plotted (b) at 2.6 K for a thermal initial state and (c) at 2.7 K with a hyperpolarized initial state. The minimum bound for each macrorealist approach is also plotted: blue for moderate, red for adversarial. Error bars represent uncertainty in measurement of the final state, and the grey point and error bars are the result of correcting for known measurement errors (namely the population damping effects of the tomography pulse sequence). The correlator sequences applied to this system are shown in Figure 3a . The final measurement at the end of an individual correlator sequence is accomplished through population tomography [20] . Figure 3: Experimental values for the LG function are compared with bounds from quantum mechanics and macrorealist theories. ( a ) The populations of the four system-ancilla (nucleus–electron) states are manipulated with microwave and radio-frequency radiation. The experimentally determined value of the Leggett–Garg function at a static field of B =3.357 T is plotted ( b ) at 2.6 K for a thermal initial state and ( c ) at 2.7 K with a hyperpolarized initial state. The minimum bound for each macrorealist approach is also plotted: blue for moderate, red for adversarial. Error bars represent uncertainty in measurement of the final state, and the grey point and error bars are the result of correcting for known measurement errors (namely the population damping effects of the tomography pulse sequence). Full size image Inequality violation We performed two experimental tests with results shown in Figure 3b,c . The first used a simple state in thermal equilibrium at 2.6 K with , yielding f =−0.031. The second used an established hyperpolarization sequence [20] from an initial state at 2.7 K. Due to the conditional nature of U this technique reduces the venality (please see Supplementary Methods ) to , yielding f =−0.296. In the course of our experiments, the fidelity of the final state populations with respect to the ideal target was never <98.9%. Our analysis has made two assumptions about the measurement process: first, that any detector imperfections do not conspire to favour anti-correlations preferentially. Second, as discussed earlier, that our null measurements do not influence the correlations through some hidden structure of the macrorealist's state. Our results then constitute a falsification of MR ∩ NIM for cold nuclear spins. Our approach relies upon the 'ideal negative result' measurements originally envisaged by LG; we show that such measurements are possible through an ancilla. Recognizing that ancilla preparation will always be imperfect, we account for the implications through a quantity termed 'venality'. We show that for sufficiently low venality even an 'adversarial' macrorealist must concede that his view is inconsistent with experimental results. Importantly this approach allows one to employ either individually controlled systems or a spatial ensemble, and it is applicable to systems of any size. For our chosen experimental system, an ensemble of phosphorous impurities in silicon, we were able to reach a low-temperature, high-field regime where the venality is low enough for our LG test to be feasible. Through the use of high-precision control techniques, we were indeed able to obtain a result representing an unequivocal violation of the inequality. The violation of this bound has secured the following profound conclusion: All accurate descriptions of systems of this type must include a concept similar to that of quantum superposition, and/or an exotic notion of measurement similar to that of wavefunction collapse. Although our experimental results relate to a microscopic system, we emphasize that our protocol is entirely general in terms of the scale of the system and whether it is individually controlled. Thus we hope that our work will give rise to a series of experiments, which probe successively more macroscopic entities with the same rigour that we apply here. Ultimately such experiments will realize Leggett and Garg's vision of establishing whether superpositions of macroscopically distinct states are indeed possible. Weak measurements versus ideal negative result measurements LG tests employ the concept of non-invasive measurement in a fundamental way; the approaches one may take when seeking an implementation include weak measurement or ideal negative result measurement. Weak measurements are likely to be regarded by both the quantum physicist and the macrorealist as approximations to true non-invasiveness. Meanwhile Leggett's concept of negative result measurement seems highly invasive to a quantum physicist but entirely non-invasive to a macrorealist. As we are interested in a test involving a gap between the predictions of quantum physics versus macrorealist theories, it is the latter approach that is preferable. The weak measurement approach cannot be altered to take account of the amount of invasiveness by defining something like the venality (which is a measure of how often a non-ideal measurement is applied and not a measure of the invasiveness of a given measurement). A back action is imparted for each and every run of the experiment, and hence the so-called 'clumsiness loophole' [12] cannot be closed this way. Sample preparation Si:P consists of an electron spin S =1/2 ( g =1.9987) coupled to the nuclear spin I =1/2 of 31 P through an isotropic hyperfine coupling of a =4.19 mT. The W-band electron paramagnetic resonance (EPR) signal comprises of two lines (one for each nuclear spin projection M I =±1/2). Our experiments were performed on the low-field line of the EPR doublet corresponding to M I =1/2. At 2.6 K and 3.36 T, the electron and nuclear spin T 1 were measured to be ∼ 1 s and 100 s, respectively. The sample consists of a 28 Si-enriched single crystal about 0.5 mm in diameter with a residual 29 Si concentration of order 70 p.p.m., produced by decomposing isotopically enriched silane in a recirculating reactor to produce poly-Si rods, followed by floating zone crystallization. Phosphorus doping of ∼ 10 14 cm −3 was achieved by adding dilute PH 3 gas to the Ar ambient during the final float zone single crystal growth. Further information on the sample growth has been reported elsewhere [21] . Pulsed EPR experiments were performed using a W-band (94 GHz) Bruker Elexsys 680 spectrometer equipped with a 6 T superconducting magnet and a low-temperature helium-flow cryostat (Oxford CF935). The cryostat was pumped to achieve a temperature of 2.6 K (internal thermocouple). Typical pulse times were 56 ns (288 ns) for a MW1 (MW2) π pulse and 90 μ s for an RF π pulse. Spin resonance experiments Both the conditional nuclear operation, and also the non-invasiveness of the measurement operation performed by the ancilla electron spin, require that the magnetic resonance pulses are selective to a high degree. The electron and nuclear spin resonance frequencies are separated by ∼ 10 and ∼ 10 4 times the pulse excitation bandwidth, respectively, hence we may rule out excitation of non-resonant spin transitions (please see Supplementary Methods ). The spin-relaxation lifetimes at 2.6 K are orders of magnitude longer than the total experiment time of 450 ms, and hence we expect (and observe) no population shifts due to relaxation on these timescales. The Leggett–Garg function f is a linear combination of populations, which can be considered as diagonal entries in a density matrix. Using magnetic resonance, only population differences can be measured. This leads to an 'observable' (or 'pseudopure') component, which can be manipulated by an experimentalist, and an 'unobservable' component, made up of populations common to all eigenstates. For each of the six subexperiments, a four dimensional 'pseudopure' matrix was measured, which was then added to an appropriately scaled identity component determined by the local magnetic field and temperature of the sample (representing the unmeasurable component of the ensemble). A baseline measurement was taken as an average of 2,000 samples, and all data sets were baseline-corrected before processing. The population differences were measured by an average of 200 samples and scaled with respect to a measured thermal amplitude (also taken as an average over 200 samples), and adjusted to have unit trace with the addition of an appropriately scaled identity matrix. Error analysis The errors corresponding to each population were calculated according to the s.e. of the direct difference measurements. These population errors were transformed into final Leggett–Garg function uncertainty by a Monte Carlo generation of density matrices. The generated matrices deviated from the measured matrix in each element by an amount chosen randomly from a normal distribution whose s.d. matched that element's error. Once re-normalized, unphysical matrices were discarded and statistics on physical matrices were collected. In total, 2 12 matrices were used to compile the final uncertainty. This constituted the 'raw' pseudopure matrix. The principal source of error in the population difference measurements came from microwave and radio-frequency inhomogeneity leading to a spread in applied rotation angles across the ensemble. These errors constituted a loss of signal for every applied pulse, with a negligible net over or underrotation. We fit the Rabi oscillations of each of the two microwave-frequency rotations and the radio-frequency rotations to arrive at an estimate for the signal lost per applied π rotation in the population tomography sequence. These fits were used to estimate the populations without the amplitude-dampening effects of the tomography sequence, and the uncertainties of these fits were used to estimate the uncertainty of each population element. These uncertainties were combined with the measurement uncertainty error before performing Monte Carlo simulations as above with 2 12 matrices. This enables us to correct for the limitations of the tomography sequence and infer the actual populations before the tomography is applied. The calculated pseudopure matrix ρ pp was added to the appropriate amount of identity matrix I as determined by the sample temperature. The explicit reconstruction is given by The diagonal entries of six matrices of this kind were used to generate each of the datapoints shown in Figure 3 . The value for f calculated from raw populations is shown there in black and the value for f calculated from populations corrected to compensate for the principal tomography errors is shown in grey, for both the hyperpolarized and un-hyperpolarized data sets. There are two conventional measures of state fidelity, or alternatively the more generous measure . When applied to physically allowed states, both measures are non-negative and reach a maximum value of 1 when ρ 1 = ρ 2 . The fidelity used in the main text calculates when comparing the gathered density matrix with the target density matrices. 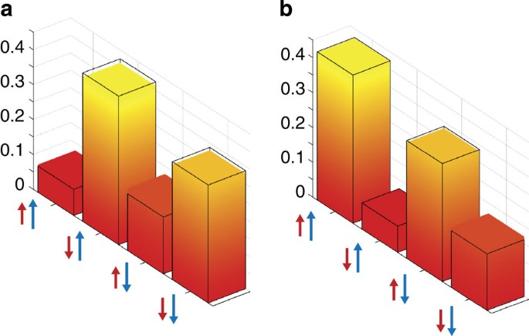Figure 4: An example of the measured populations acquired from tomography. Orange bars represent diagonal matrix elements at the end of the second core experiment. The wireframes are the ideal quantum values. The populations were acquired froma, the cnot circuit andb, the anti-cnot circuit. Examples of gathered versus ideal populations are shown in Figure 4 . Figure 4: An example of the measured populations acquired from tomography. Orange bars represent diagonal matrix elements at the end of the second core experiment. The wireframes are the ideal quantum values. The populations were acquired from a , the cnot circuit and b , the anti-cnot circuit. Full size image How to cite this article: Knee, G. C. et al . Violation of a Leggett–Garg inequality with ideal non-invasive measurements. Nat. Commun. 3:606 doi: 10.1038/ncomms1614 (2012).